Selective anion exchange with nanogated isoreticular positive metal-organic frameworks Crystalline porous materials, especially inorganic porous solids such as zeolites, usually have negative frameworks with extra-framework mobile cations and are widely used for cation exchange. It is highly desirable to develop new materials with positive frameworks for selective anion exchange and separation or storage and delivery. Recent advances in metal-organic framework synthesis have created new opportunities in this direction. Here we report the synthesis of a series of positive indium metal-organic frameworks and their utilization as a platform for the anion exchange-based separation process. This process is capable of size- or charge-selective ion-exchange of organic dyes and may form the basis for size-selective ion chromatography. Ion-exchange dynamics of a series of organic dyes and their selective encapsulation and release are also studied, highlighting the advantages of metal-organic framework compositions for designing host materials tailored for applications in anion separation and purification. Metal-organic frameworks (MOFs) have been recognized as an excellent platform for host-guest chemistry, which includes gas storage [1] , [2] , [3] , [4] , [5] , ion-exchange [6] , [7] , [8] , [9] , [10] , separation [11] , [12] , [13] , [14] , [15] , [16] , and so on [17] , [18] , [19] , [20] , [21] , [22] , [23] . The pore size of MOFs varies from a few angstroms to a few nanometres, making them ideal for incorporating species ranging from small gas molecules [24] , [25] , [26] and organic molecules [27] , [28] to large inorganic and organic species [29] , [30] , [31] , [32] . Although the adsorption and separation of gas molecules [11] and small organic molecules [12] , [13] , [14] , [28] (limited to one benzene ring, Mw<100 Da) have been extensively studied, the incorporation and separation of bulky molecules (~100 Da<Mw<~1,000 Da), especially anionic, have been much less reported [15] . The separation of organic species at this size level has great practical significance in biotechnology and pharmaceutical industry, because of the need for the separation of peptides, nucleotides, amino acids, drug molecules, and so on. The incorporation and controlled release of organic species at this size level is also relevant to drug delivery [21] . Currently, ion-exchange chromatography and ion-exchange solid phase extraction based on ion-exchange resins are known as powerful tools for the separation of charged molecules. The strong coulombic interaction between the charged stationary phase and analytes contributes to the high efficiency and sensitivity of the separation process. Another separation method, size-exclusion chromatography, is based on size or molecular weight of the analytes and is especially useful for the separation of very large species, such as proteins and polymers. By combining the unique structural features of MOFs and the efficiency of ion chromatography, it is possible to develop a novel separation system, in which charged MOFs replace the conventional ion-exchange resins as the separation medium ( Fig. 1 ). The structural characteristics of MOFs such as the precisely defined pore, and window size tunable with reticular synthesis can result in useful properties such as size-exclusion effect for guest molecules in a size regime that cannot be achieved by conventional ion-exchange resins. 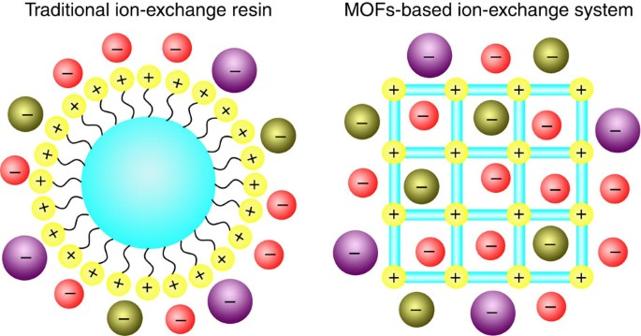Figure 1: Ion-exchange resin versus MOFs as ion-exchange medium. Comparison between traditional ion-exchange resin (left) and MOFs based ion-exchange systems (right) for ion chromatography. The red, greenish and purple balls with ‘−’ signs represent mobile guest anions in different sizes. Figure 1: Ion-exchange resin versus MOFs as ion-exchange medium. Comparison between traditional ion-exchange resin (left) and MOFs based ion-exchange systems (right) for ion chromatography. The red, greenish and purple balls with ‘−’ signs represent mobile guest anions in different sizes. Full size image So far, there have been limited studies on ion-exchange-based separation processes with MOFs. Although ion-exchange of small or bulky guest species into charged frameworks has been observed [6] , [7] , [8] , [9] , [10] , [31] , most of the studies were focused on the capture of specific metal ions [6] , [7] or the enhancement of gas-sorption capability [8] . There are also examples of liquid chromatography for organic dyes using Zn MOFs with neutral framework [33] , [34] , [35] , which are less likely to involve ion-exchange. Depending on the charge of analyte, both negative and positive stationary phases are desired for ion chromatography. Here we are particularly interested in the separation of organic anions. Among reported MOFs, there are comparatively few permanently porous MOFs with positive framework (P-MOFs) [6] , [36] , [37] , whose rarity is also mirrored in other types of porous materials, including zeolites [38] , [39] , [40] , [41] , [42] , [43] , [44] , [45] . In addition, known P-MOFs often have low stability or small pore size that only permits the exchange of small inorganic anions [7] , [10] . Therefore, the construction of P-MOFs with tunable open architecture that will allow for the exchange and separation of bulky anions is highly desirable. Here we report the systematic synthesis of P-MOFs using positive secondary building units. Specifically, a family of [In 3 O(COO) 6 ] + -based P-MOFs have been made and used as the platform to study the ion-exchange-based separation process. The charge- and size-dependent ion-exchange dynamics of a series of organic dyes are demonstrated. Synthesis of trimer-based P-MOFs Methods for creating P-MOFs include combining metal ions with neutral ligands or introducing positive secondary building units into the framework. The latter strategy is adopted here, because it generally leads to the frameworks with higher stability owing to the higher connectivity and stronger node-linker bonds. In MOFs, the trimer in the form of M 3 O[COO] 6 or M 3 (OH)[COO] 6 is well known. Its charge can be neutral or positive, depending on the charge of metal ions (+3 or mixed +3/+2) and the charge of ligands (0 or −1) at the three axial positions ( Supplementary Fig. S1 ). For example, the Ni II 2 Ni III (OH)(COO) 6 is neutral due to the mixed valence of Ni and the central μ 3 -OH [46] , [47] , [48] . In contrast, [In 3 O(COO) 6 ] + is positive when all of its three axial positions are occupied by neutral groups. If, however, one axial position is capped with a negative species such as OH − , the cluster becomes neutral. Thus to generate P-MOFs, it is important to prevent any possibility of having a negative dangling ligand such as F − on the cluster. For this reason, a recently reported 9-connected ncb net originally obtained as neutral Ni MOFs was selected as our target topology [46] , [47] , [48] . In the ncb net, all three axial sites of the trimer are occupied by the pyridyl groups. By using the positive indium trimers to replace the neutral nickel trimers, the overall framework becomes positive. The indium trimer-based cationic frameworks (ITCs) contain two different types of linear ditopic ligands, the mono-negative isonicotinate type ligand ( L1 , including isonicotinate (ina), 4-(pyridine-4-yl)benzoate (pba)) and the di-negative terephthalate type ligand ( L2 , including terephthalate (bdc), 2-aminoterephthalate (NH 2 -bdc), 2-bromoterephthalate, 2,6-naphthalenedicarboxylate (ndc) and 4,4′-biphenyldicarboxylate (bpdc)) in a 2:1 molar ratio ( Fig. 2a ). By applying different combinations of L1 and L2 , six isostructured ITCs were obtained ( Supplementary Table S1 ). 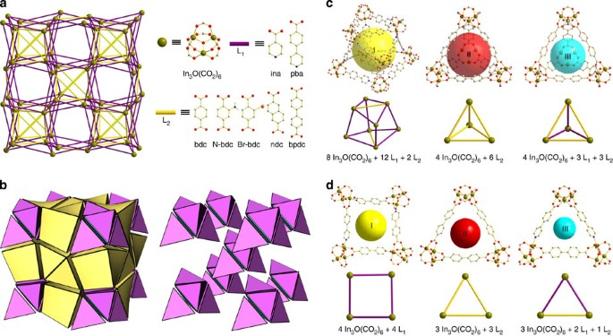Figure 2: Structural features of ITC-n. (a) The 9-connectedncbnet topology constructed from one type of node (In3O trimer) and two types of linear edges (purple L1 and yellow L2 ligands). (b) the tiling diagrams showing three types of tiles and the NbO type channel system (the space filled with yellow tiles). (c) three types of pores and their building units. (d) three types of windows and their building units. ina=isonicotinate; pba=4-(pyridine-4-yl)benzoate; bdc=terephthalate; N-bdc=2-aminoterephthalate; Br-bdc=2-bromoterephthalate; ndc=2,6-naphthalenedicarboxylate; and bpdc=4,4′-biphenyldicarboxylate. Figure 2: Structural features of ITC-n. ( a ) The 9-connected ncb net topology constructed from one type of node (In 3 O trimer) and two types of linear edges (purple L1 and yellow L2 ligands). ( b ) the tiling diagrams showing three types of tiles and the NbO type channel system (the space filled with yellow tiles). ( c ) three types of pores and their building units. ( d ) three types of windows and their building units. ina=isonicotinate; pba=4-(pyridine-4-yl)benzoate; bdc=terephthalate; N-bdc=2-aminoterephthalate; Br-bdc=2-bromoterephthalate; ndc=2,6-naphthalenedicarboxylate; and bpdc=4,4′-biphenyldicarboxylate. Full size image Pore structure control and analysis The structures of ITCs were determined using single-crystal X-ray crystallography ( Supplementary Figs S13–S17 and Supplementary Tables S3–S7 ), and all have the same ncb topology. This topology, featuring a 9-connected indium trimer, was first reported for Ni by Chen and Zhang et al. [46] , [47] , [48] Although there are quite a few examples of frameworks based on 6-connected indium trimers, higher-connected indium trimers such as those reported here are much less observed. Before this work, an 8-connected indium-trimer-based framework was reported by Xu et al. [49] Coincidentally, Xu’s framework is also constructed from L1 to L2 type ligands, yet in a 1:1 molar ratio. The reason for the occurrence of these two 9- and 8-connected structures may lie in the different length ratio between L1 and L2 . Xu’s structure features a short L1 ligand (isonicotinic acid) and a long L2 ligand (4,4′-azodibenzoic acid), whereas in the ncb structures, the length of L1 and L2 is much closer, although there is considerable flexibility in the length range for L2 when pba was used for L1 . Here the structure contains three types of cages ( Fig. 2c ), named cage I, II and III. Cage I is a distorted cube-like cage constructed from 8 indium trimers, 12 L1 and 2 L2 , and cage II is an equilateral tetrahedron constructed from 4 trimers and 6 L2 , whereas cage III is an irregular tetrahedron constructed from 4 trimers, 3 L1 and 3 L2 . Cage I is interconnected with each other to form an NbO type three-dimensional channel system (Fig. 2b ), which is responsible for the largest portion of the void space within the framework. To evaluate the accessibility of organic molecules to the voids of the frameworks, both window size and pore size need to be considered. The window size is responsible for the size selectivity of guest species, whereas the pore size defines the volume available for the guest and affects the ion-exchange capacity. We analysed and summarized the dimensional information for both pores and windows for all the six structures ( Supplementary Fig. S5 and Supplementary Table S2 ). It is found that although the three types of cages are associated with three types of pores ( Fig. 2c ) and three types of windows ( Fig. 2d ), the dimensions of the type I pore and window are larger than others. Thus, they are expected to have greater impact on the ion-exchange process and should be taken into primary consideration. In particular, the type I window will provide the size selectivity and contribute most to the exchange dynamics. Type II and III pores and windows may also have some effects on exchange rate and capacities. Anionic organic dyes as the model guest Here owing to their appropriate molecular mass (at the 100–1,000 Da level) and the ease of detection, organic dyes are selected as guest molecules to study ion-exchange properties. To exclude other possible effects due to differences in guest molecules, a series of azo type dyes with similar backbone but different charges and sizes are selected ( Table 1 and Supplementary Fig. S6 ). Although the charge is easily varied by the number of sulphonate group, the variation in size is more complicated because it involves both dimension and molecular weight. The dimension will affect both the accessibility to the pore and the exchange dynamics, whereas the molecular weight mainly affects the dynamics. To estimate the accessibility of organic dyes to the pore, the dimensions of the organic dyes are defined as x × y × z ( x ≤ y ≤ z ), wherein x , y and z are the three edges of a cuboid that can just include the molecule, and they are chosen to make y as small as possible (the smallest second minimum dimension, or MIN-2). With such definition, MIN-2 becomes the most important parameter for estimating the size of guest molecule relative to the window size of the host. Table 1 Molecular weight and dimensions of guest dye molecules with different charges. Full size table Charge and size of the guest are the two most important factors during the ion-exchange process. We have arranged the organic dyes in two groups. Dyes in the first group have different charges, but similar size (Methylene blue, MLB + ; Sudan I, SDI 0 ; acid orange 7, AO7 − ; orange G, OG 2 − ; and new coccine, NC 3 − ), whereas dyes in the second group have different size, but the same charge ( OG 2 − ; Ponceau 6R, P6R 2 − ; Croscein scarlet 3B, CS3B 2 − ; Croscein scarlet 7B, CS7B 2 − ; acid black 1, AB1 2 − ; and methyl blue, MB 2 − ). The ion-exchange experiments of individual dye solutions are then performed on P-MOFs including ITC-4 ( Supplementary Figs S7–S10 ), ITC-1 ( Supplementary Fig. S11a ), ITC-2 series ( Supplementary Fig. S11d–f ), ITC-3 ( Supplementary Fig. S11g ) and neutral host Ni-MOFs (ITC-2-Ni and ITC-3-Ni) ( Supplementary Fig. S11b,c ). The separation process based on size- and charge-selective ion-exchange is further demonstrated in the solutions containing two different dyes. Selectivity for anionic dyes by P-MOF A cationic dye ( MLB + ) and an anionic dye ( OG 2 − ) were chosen as guests to make a mixture because they have opposite charge but their sizes are relatively small and close to each other, so that the size effect can be excluded. A light orange solution of OG 2 − and a light blue solution of MLB + were mixed thoroughly to give a green coloured solution of equimolar mixture. Then this solution was transferred to a vial containing ITC-4. The colour of the solution gradually turned blue from green and essentially came to a colour that was the same as the pure MLB + solution after about 2 days. Meanwhile, the original white ITC-4 powder at the bottom of the vial became orange ( Fig. 3a ), an indication of trapping of the anionic dye OG 2 − within the pore. The above observation was also proved by the UV–vis spectroscopy. The result indicated that only the anionic guest could enter ITC-4 and the cationic guest was denied access. 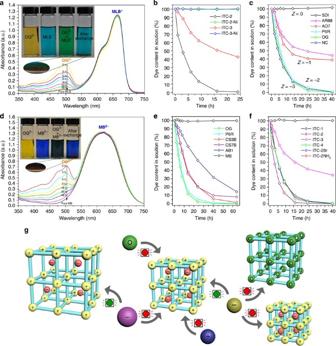Figure 3: Size and charge selectivity and ion-exchange dynamics. (a) UV–vis spectra of equimolarOG2−andMLB+mixture in the presence of ITC-4, monitored with time. The photographs show the colours ofOG2−andMLB+solutions, their mixture before and after ion-exchange for 48 h. The photograph below the vials shows the solid with the orange colour. (b) Percentage ofOG2−remaining in the solution monitored with time. (c) Percentage of differently charged dyes remaining in the solution monitored with time in the presence of ITC-4. (d) UV–vis spectra of equimolarOG2−andMB2−mixture in the presence of ITC-4, monitored with time. The photographs show the colour ofOG2−andMB2−solution, their mixture before and after ion-exchange for 48 h and the photograph below the vials shows the solid with the orange colour ofOG2−. (e) Percentage of differently sized dyes (−2 charged) remaining in the solution monitored with time in the presence of ITC-4. (f) Percentage ofOG2−remaining in the solution monitored with time in the presence of six isoreticular MOFs with different L1 and L2. (g) The schematic illustration of the ion-exchange process. Frameworks with yellow nodes represent P-MOFs with three different pore sizes and the framework with green nodes represents the neutral host with same topology. Red spheres with ‘−’ represent the original NO3−counter ions and the purple, blue, green and golden spheres labelled with ‘+, −, or 0’ represent organic guests with different charges and sizes. Arrows show whether a given ion-exchange process is permissible or non-permissible due to size or charge exclusion. Flashing green circles mean the exchange process is allowed, while flashing red circles mean that the process is disallowed. Figure 3: Size and charge selectivity and ion-exchange dynamics. ( a ) UV–vis spectra of equimolar OG 2− and MLB + mixture in the presence of ITC-4, monitored with time. The photographs show the colours of OG 2− and MLB + solutions, their mixture before and after ion-exchange for 48 h. The photograph below the vials shows the solid with the orange colour. ( b ) Percentage of OG 2− remaining in the solution monitored with time. ( c ) Percentage of differently charged dyes remaining in the solution monitored with time in the presence of ITC-4. ( d ) UV–vis spectra of equimolar OG 2− and MB 2− mixture in the presence of ITC-4, monitored with time. The photographs show the colour of OG 2− and MB 2− solution, their mixture before and after ion-exchange for 48 h and the photograph below the vials shows the solid with the orange colour of OG 2− . ( e ) Percentage of differently sized dyes (−2 charged) remaining in the solution monitored with time in the presence of ITC-4. ( f ) Percentage of OG 2− remaining in the solution monitored with time in the presence of six isoreticular MOFs with different L1 and L2. ( g ) The schematic illustration of the ion-exchange process. Frameworks with yellow nodes represent P-MOFs with three different pore sizes and the framework with green nodes represents the neutral host with same topology. Red spheres with ‘−’ represent the original NO 3 − counter ions and the purple, blue, green and golden spheres labelled with ‘+, −, or 0’ represent organic guests with different charges and sizes. Arrows show whether a given ion-exchange process is permissible or non-permissible due to size or charge exclusion. Flashing green circles mean the exchange process is allowed, while flashing red circles mean that the process is disallowed. Full size image Selectivity for P-MOF by anionic dyes We also tested the response of the same anionic dye to neutral and positive MOFs. To make the results comparable, effects other than the charge of the framework need to be minimized. Thus, materials with the same structure but different charge are desired. Here we were able to synthesize two neutral Ni compounds (ITC-2-Ni and ITC-3-Ni) isostructural with positive indium-based ITC-2 and ITC-3 ( Supplementary Fig. S1 ). The anion exchange experiments were performed under the same condition for all four MOFs with OG 2 − as the anionic guest. The results show that although the dye concentrations in ITC-2 and ITC-3 dropped dramatically with time, the dye concentrations in ITC-2-Ni and ITC-3-Ni stayed constant ( Fig. 3b ). This observation indicated that the OG 2 − anions were gradually exchanged into the cationic frameworks of ITC-2 and ITC-3, but were not able to enter the neutral frameworks of ITC-2-Ni and ITC-3-Ni. Such results again clearly demonstrate the primary role of coulombic interaction in such a process. Charge dependency of ion-exchange dynamics Although the charge selectivity described above shows that the ion-exchange process is forbidden when host and guest are not charge complementary, it is also interesting to determine how the ion-exchange dynamics can be affected by the magnitude of charge. Thus, we studied the ion-exchange process of a series of differently charged dyes upon the same ITC-4 platform ( Fig. 3c ). To make the experimental results comparable, a series of azo type dyes ( SDI 0 , AR88 − , AO7 − , OG 2 − , P6R 2 − and NC 3 − , see Table 1 ) with similar backbone, size and molecular weight, but different charge were chosen. The ion-exchange results after a period of 40 h showed that although the concentration of the anionic AR88 − , AO7 − , OG 2 − , P6R 2 − and NC 3 − decreased to different extent, the concentration of the neutral SDI 0 stayed constant. Such observation again indicates that the ion-exchange process is charge-selective and even the neutral species cannot diffuse into the P-MOF. More importantly, their ion-exchange rates were found to be dependent on the magnitude of the charge. The exchange rates of −1-charged AR88 − and AO7 − are the slowest, yet close to each other. In contrast, the ion exchange of −2-charged OG 2 − and P6R 2 − is faster and so is −3-charged NC 3 − . In addition, although the ion exchange of the −2-charged OG 2 − , P6R 2 − and −3-charged NC 3 − is complete, the ion-exchange of −1-charged AR88 − and AO7 − is incomplete, with their concentration becoming almost constant after 40 h. It is necessary to point out that the molecular mass of the dyes becomes larger with increasing charge, which may have the opposite effect on the ion-exchange rate. This could explain the less obvious difference between NC 3 − and OG 2 − . Size-exclusion effect To demonstrate size dependency, the ion-exchange behaviour of equimolar mixture of OG 2 − and MB 2 − was monitored in the presence of ITC-4. OG 2 − and MB 2 − are chosen as they are significantly different in size but have the same −2 charge. The mixing of light orange coloured OG 2 − solution and the deep blue coloured MB 2 − solution gave a dark slate grey coloured solution, which was transferred to a vial containing ITC-4 and was monitored by UV–vis periodically ( Fig. 3d ). The colour of the solution gradually turned bluish and finally turned to a blue colour (identical to the pure MB 2 − solution) after 2 days. At the same time, the white ITC-4 powder turned to a deep orange colour due to the trapping of OG 2 − inside the pores. This observation is supported by the UV–vis measurements. To ensure such selectivity is not a result of dynamic competition between the above two anions, the ion-exchange process of MB 2 − was examined individually, which showed that MB 2 − was indeed denied access by ITC-4 ( Fig. 3e ). Dependency of ion-exchange dynamics on size of dyes A series of anionic dyes with different sizes were chosen to study their ion-exchange processes in parallel ( OG 2 − , P6R 2 − , CS3B 2 − , CS7B 2 − and AB1 2 − , see Table 1 ) with ITC-4 as the host. The charges of the anionic guests are kept the same ( Z =−2) to minimize the difference in coulomb interaction. In the sequence given above, their molecular weights, as well as dimensions, gradually increase. The ion-exchange result after a period of 64 h showed that different from MB 2 − , all the five dyes can be exchanged into ITC-4 to different extent ( Fig. 3e ). More importantly, their ion-exchange dynamics are different and related to their dimensions and molecular weights. In general, the ion-exchange processes become slower with increasing size of the guest. Notably, as OG 2− and P6R 2− are similar to each other in molecular weight and dimension, their ion-exchange dynamics are close to each other, and so are CS3B 2− and CS7B 2− . These observations indicate that the size difference provides an additional basis for separation by ion-exchange, in addition to the charge difference. Dependency of ion-exchange dynamics on pore size The size effect was also studied by applying the same guest ( OG 2− in this work) on six isoreticular structures with varied pore properties resulting from different combinations of L1 and L2 ( Supplementary Table S1 ). The results showed that although OG 2− was unable to access the pore of ITC-1, it could be exchanged into the other five structures but at different rate ( Fig. 3f ). These results indicate that the length of L1 ligand is mainly responsible for the size-exclusion effect, whereas the length of L2 ligand contributes to differing dynamics of ion-exchange. The overall ion-exchange process is depicted in Fig. 3g . It is shown that only charge and size compatible ions can be exchanged into P-MOFs. Such size and charge selectivity provides a useful basis for the design of ion-exchange systems, especially for the separation and purification of anionic species. Controlled release and recyclability In practical use, the reversibility of the ion-exchange process is required. The reversibility is also relevant to drug delivery. The ion-exchange process is intrinsically reversible as it is based on the dynamic equilibrium between different guests, which can be shifted by relative concentrations. In this work, the release experiment was performed following the ion-exchange process in which OG 2− had been fully loaded into ITC-4 ( Fig. 4a ). At the end of the ion-exchange, the solution turned colourless from the initial orange colour, as OG 2− was removed from the solution by ion-exchange into the MOF solid, which turned orange from white due to the trapping of OG 2− . With the replacement of the upper colourless solution by the same volume of solution containing NaNO 3 , the release process was triggered. The colour of the solution turned back to orange as OG 2− was displaced from the MOF by nitrate anions through ion-exchange, and the powder turned back to white again. The UV–vis measurement showed that the release of OG 2− was almost 100% after 12 h. Such an ion-exchange and release process was performed for 10 continuous cycles, and the process is entirely reversible with no observable drop in the ion-exchange capacity ( Fig. 4b ). The powder X-ray diffraction of ITC-4 after 10 exchange-release cycles showed the same pattern as before, indicating the high stability of the host material ( Fig. 4d ). 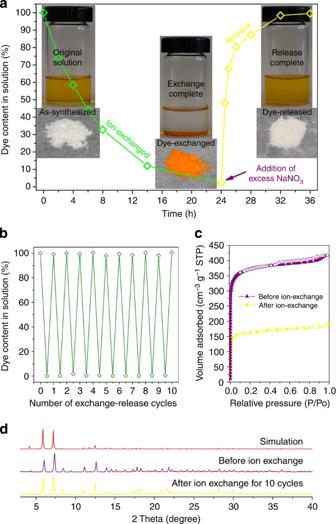Figure 4: Reversibility and recyclability for ion-exchange. (a) The reversible trapping and releasing of the dye in a full ion-exchange and release cycle. The release is triggered by the addition of excess NaNO3. (b) The dye concentration monitored for 10 exchange-release cycles. (c) N2sorption isotherms (at 77 K) of ITC-4 before and after ion-exchange with a 2:1 MOF toOG2−ratio. (d) Experimental powder XRD pattern of ITC-4 before and after ion-exchange for 10 cycles, compared with the simulated pattern. Figure 4: Reversibility and recyclability for ion-exchange. ( a ) The reversible trapping and releasing of the dye in a full ion-exchange and release cycle. The release is triggered by the addition of excess NaNO 3 . ( b ) The dye concentration monitored for 10 exchange-release cycles. ( c ) N 2 sorption isotherms (at 77 K) of ITC-4 before and after ion-exchange with a 2:1 MOF to OG 2− ratio. ( d ) Experimental powder XRD pattern of ITC-4 before and after ion-exchange for 10 cycles, compared with the simulated pattern. Full size image Ion-exchange capacity In the previous experiments, the concentration of dye was kept low (MOF:dye=20:1 in molar ratio, the MOF formula unit is based on one In 3 O trimer and one NO 3 − ) to make it within the detectable range of UV–vis measurements as well as to reduce the time for the ion-exchange process. Although a medium-sized dye such as OG 2− can be fully exchanged into the MOF under such low-concentration conditions, it is interesting to find out the amount of dye that can be loaded into the host when the dye concentration is high. Thus, the ion-exchange experiment was also performed with the concentration of OG 2− raised by 10-fold (MOF:dye=2:1 in molar ratio, 2NO 3 − per OG 2− ). The result showed that about 47.2% of the NO 3 − in ITC-4 was replaced by OG 2− when the ion-exchange reached the equilibrium after 4 days. It is reasonable to expect an even higher capacity when an additional amount of OG 2− is applied to shift the equilibrium further. The N 2 sorption results before and after ion-exchange gave the BET surface area of 1,078 m 2 g −1 and 505 m 2 g −1 , respectively. The decrease in the BET surface area results from the decreased pore volume owing to the inclusion of OG 2− instead of NO 3 − ( Fig. 4c ). One advantage of MOF over conventional ion-exchange resin is its well-defined and uniform pore size and their size-exclusion effect at the nanometre scale. Although the size-exclusion effect has been demonstrated here, it is generally difficult to predict whether a given guest is able to access a certain host due to the irregular and varied shape of the guests and the complexity of the pore system, especially when their dynamic models are taken into consideration. Here we propose a simple method to analyse and estimate the accessibility. Instead of using sophisticated calculations based on dynamic models, the static structural models are used for the analysis of both window size and guest size, which is much simpler but can still give a useful model. In this method, two window dimensions are defined. The lower limit of the window size is defined as d min , which is usually the diameter of the maximum fit circle ( Fig. 5a ) and the upper limit of the window size is defined as d max , which is usually related to the shape of window. In this specific case, d max is the diagonal length of the maximum fit square ( Fig. 5b ). The size of a guest molecule is defined using a cuboid model as described previously ( Fig. 5c ). When MIN-2>d max , the access of guest to the pore is not possible, and when MIN-2<d min , the access of guest to the pore is allowed ( Fig. 5d ). When d min <MIN-2<d max , the accessibilty depends on its shape. When both guest and host are given, a chart can be made to help understand the observed size-exclusion. For example, the MIN-2 of OG 2− (10.14 Å) is larger than the d max of ITC-1 (7.2 Å) ( Fig. 5d ), which explains why the OG 2− is blocked by ITC-1 ( Supplementary Fig. S11a ). Similarly, MB 2− (MIN-2 as 14.35 Å) cannot enter ITC-4 (d max as 12.1 Å) due to its relatively larger size ( Fig. 3d ). In comparison, the MIN-2 of OG 2− (10.14 Å) and AB1 2− (11.15 Å) are between d min (7.8 Å) and d max (12.1 Å) of ITC-4, they are able to enter ITC-4, due to their relatively small x dimension (~5.5 Å). 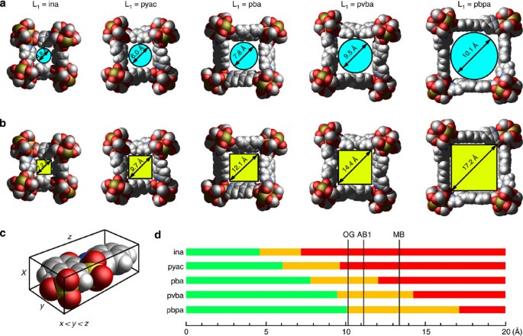Figure 5: Analysis of type I windows in five isoreticular structures. (a) dmindefined by the diameter of the largest fit circle, which is the lower limit of the window size. (b) dmaxdefined by the diagonal length of the largest fit square, which is the upper limit of the window size. (c) the dimension of a guest molecule defined by the cuboid model;x,y,zare chosen to makex<y<zand y as small as possible. (d) a bar chart revealing the dminand dmaxof five isoreticular structures. A guest molecule withy<dminis allowed by the window (green), whereas a guest molecule withy>dmaxis excluded by the window (red), when dmin<y<dmax, the accessibility of guest molecule depends on its shape (yellow). pyac=(E)-3(pyridine-4-yl)acrylate; pvba=(E)-4-(2-(pyridine-4yl)vinyl)benzoate; and pbpa=4′-(pyridine-4-yl)biphenyl-5-carboxylate. Figure 5: Analysis of type I windows in five isoreticular structures. ( a ) d min defined by the diameter of the largest fit circle, which is the lower limit of the window size. ( b ) d max defined by the diagonal length of the largest fit square, which is the upper limit of the window size. ( c ) the dimension of a guest molecule defined by the cuboid model; x , y , z are chosen to make x < y < z and y as small as possible. ( d ) a bar chart revealing the d min and d max of five isoreticular structures. A guest molecule with y <d min is allowed by the window (green), whereas a guest molecule with y >d max is excluded by the window (red), when d min < y <d max , the accessibility of guest molecule depends on its shape (yellow). pyac=(E)-3(pyridine-4-yl)acrylate; pvba=(E)-4-(2-(pyridine-4yl)vinyl)benzoate; and pbpa=4′-(pyridine-4-yl)biphenyl-5-carboxylate. Full size image The guest molecules of different sizes and shapes can be further distinguished through synthetic design of P-MOFs with different window and pore sizes. For a given guest, the access control can be achieved by the host selection, based on the need of each specific application. As an example, a series of isoreticular structures are illustrated here ( Fig. 5 ), and they give a set of continuously variable pore properties. From the above experiments, it is known that the type I pore has the largest effect on the ion-exchange process and provides the size selectivity. Thus, in addition to ITC-1 and ITC-4, three hypothetical structures are also included, which can be realized through isoreticular synthesis (previously demonstrated by Ni structures) [46] . These five structures are varied by L1 (ina, pyac, pba, pvba and pbpa, respectively, with increasing length, Fig. 5 ), which defines the type I window. Thus, when a guest is given, the chart will help predict the ion-exchange behaviour in different hosts, and the appropriate host can be selected to control the accessibility. In conclusion, we have employed positive indium trimer [In 3 O(COO) 6 ] + for the creation of a series of pore size tunable P-MOFs and demonstrated their ion-exchange properties, which may serve as the basis for applications in ion chromatography. By using the UV–vis spectroscopy, the ion-exchange processes of organic dyes in these P-MOFs have been examined, demonstrating highly selective ion-exchange processes on the basis of charge and size of organic dyes. Even for dye molecules that can undergo ion-exchange, the ion-exchange dynamics can still differ significantly according to the magnitude of charge (−1, −2...), molecular weight, size and shape, which provides additional basis for applications in ion chromatography. Such selective anion exchange, controlled by the structural characteristics of MOFs, is advantageous and complementary to conventional ion-exchange resin, because of its suitability for molecules within ~100 Da<Mw<~1,000 Da range. Furthermore, the controlled release of guest anions make these P-MOFs potential candidates for use as drug carriers. The reticular synthesis and the large number of possible MOF structures make it possible to build an extensive library of hosts that can be used for guests (anionic in particular) of different sizes. Materials All of the reagents used were obtained from commercial supplies without further purification. In(NO 3 ) 3 ·(H 2 O) was dried overnight in the vacuum oven before use. Preparation of [In 3 O(pba) 3 (ndc) 1.5 ](NO 3 ) (ITC-3) A mixture containing In(NO 3 ) 3 ·(H 2 O) (31.9 mg, 0.1 mmol), Hpba (20.0 mg, 0.1 mmol) and H 2 ndc (11.0 mg, 0.05 mmol) was dissolved in 2.0 g DMA solution and kept at 120 o C oven for 4 days. Pure colourless truncated-cube-like crystals were obtained ( Supplementary Methods ). Preparation of [In 3 O(pba) 3 (bpdc) 1.5 ](NO 3 ) (ITC-4) A mixture containing In(NO 3 ) 3 ·(H 2 O) (31.9 mg, 0.1 mmol), Hpba (20.0 mg, 0.1 mmol) and H 2 bpdc (14.0 mg, 0.05 mmol) was dissolved in 2.0 g DMA solution and kept at 90 o C oven for 5 days. Pure colourless truncated-cube-like crystals were obtained. Measurements Single-crystal X-ray analysis ( Supplementary Data 1 ) was performed on a Bruker APEX II diffractometer with nitrogen-flow temperature controller using graphite-monochromated MoKα radiation ( λ =0.71073 Å), operating in the ω and ϕ scan mode. The SADABS programme was used for absorption correction. The structure was solved by direct methods followed by successive difference Fourier methods. All non-hydrogen atoms were refined anisotropically. Computations were performed using SHELXTL and final full-matrix refinements were against F 2 . Powder X-ray diffraction experiments were performed on a Bruker D8 Advance X-ray powder diffractometer operating at 40 kV and 40 mA (CuKα radiation, λ =1.5418 Å). The data collection were performed with a step size of 0.03° and counting time of 3 s per step. The simulated powder XRD pattern was obtained from the single-crystal data. The thermogravimetric analysis was carried out using a TA Instruments SDT Q600 apparatus in the temperature range of 30 o C to 900 o C under N 2 flow at a heating rate of 10 o C min −1 . Gas-sorption measurements were carried out on a Micromeritics ASAP 2020 Physisorption Analyser. Before the measurement, the as-synthesized sample was soaked in dichloromethane for 6 days during which period the dichloromethane bath was refreshed twice. After filtered and dried in the vacuum oven overnight, the sample was further dried by using the ‘degas’ function of the surface area analyser for 10 h at 80 o C. The N 2 sorption measurement was performed at 77 K. Ion-exchange experiments Ion-exchange experiments were performed by immersing the MOF materials in the dye/dimethylformamide (DMF) solution, which was kept still during the entire ion-exchange process. UV–vis absorbance measurements were performed periodically for the upper clear solution, which was poured back to the original system after each measurement to keep the total amount of sample constant. For most measurements, the molar ratio between MOF and dye was kept at 20:1. The absorbance maximum of original dye solution (before ion-exchange) was normalized and the percentage of dye remaining in the solution is calculated by comparing the absorbance maximum with the original dye solution. In a typical measurement, 13.8 mg (10 μmol) as-synthesized ITC-4 was weighed out to a 20 ml vial, and 6.0 g DMF solution containing 0.22 mg (0.5 μmol) Orange G was added to the vial. Then the upper clear solution was taken out for UV–vis absorbance measurement at 0 h, 2 h, 4 h, 6 h, 8 h, 14 h, 24 h, 40 h and 64 h, respectively. After each measurement, the solution was poured back to the original vial to avoid the loss of the sample. The absorbance at maximum wavelength ( λ max =503.5 nm for OG 2− ) was chosen to calculate the dye content, and the absorbance value for the original solution was normalized as 100%. The release experiment was carried out right after the completion of an ion-exchange process of OG 2− on ITC-4. It was triggered by replacing the upper clear DMF solution by the same volume of DMF solution containing 85.0 mg (1 mmol) NaNO 3 . The cycle experiments were done by performing ion-exchange, release, and filtering in turn for 10 cycles. The measurements were performed after completion of ion-exchange and release. The ion-exchange and release process was accelerated by stirring. The ion exchange capacity experiment was carried out by dissolving 11.3 mg (25 μmol) OG 2− into 10.0 g of DMF, and 68.9 mg (50 μmol) of ITC-4 was applied for the ion-exchange. Considering the −2 charge of OG 2− , the applied 2:1 molar ratio between ITC-4 and OG 2− actually gives a molar ratio of NO 3 − to RSO 3 − as 1:1 (or 50% of NO 3 − among all anions). The above OG 2− solution shows high absorbance, so solutions need to be diluted for UV–vis measurement. Stirring is used to accelerate the ion-exchange process. After a period of about 96 h, the ion-exchange process reached equilibrium. By comparing the UV–vis absorbance of the solutions before and after ion-exchange, it was calculated that approximately 13.2 μmol of OG 2− remained in the solution at the end of the ion-exchange process, which corresponds to about 47.2% of the NO 3 − being replaced by the OG 2− . How to cite this article: Zhao, X. et al. Selective anion exchange with nanogated isoreticular positive metal-organic frameworks. Nat. Commun. 4:2344 doi: 10.1038/ncomms3344 (2013).